Dual origin of defect magnetism in graphene and its reversible switching by molecular doping Control of magnetism by applied voltage is desirable for spintronics applications. Finding a suitable material remains an elusive goal, with only a few candidates found so far. Graphene is one of them and attracts interest because of its weak spin–orbit interaction, the ability to control electronic properties by the electric field effect and the possibility to introduce paramagnetic centres such as vacancies and adatoms. Here we show that the magnetism of adatoms in graphene is itinerant and can be controlled by doping, so that magnetic moments are switched on and off. The much-discussed vacancy magnetism is found to have a dual origin, with two approximately equal contributions; one from itinerant magnetism and the other from dangling bonds. Our work suggests that graphene’s spin transport can be controlled by the field effect, similar to its electronic and optical properties, and that spin diffusion can be significantly enhanced above a certain carrier density. Electric field control of magnetic properties has been the subject of considerable attention, with a few materials and hybrid magnetic systems found recently, where it is possible to control the magnetization direction and/or the Curie temperature [1] , [2] , [3] . Electric field tunability is one of the fundamental properties of graphene and has been widely used to control its electronic, optical and other properties related to the electronic structure [4] . On the other hand, graphene is believed to be an ideal material for spintronics [5] because of the weak spin–orbit interaction and long spin relaxation lengths [6] , [7] and the possibility to introduce paramagnetic centres via controlled introduction of defects, as recent experiments [8] , [9] have shown that both vacancies and adatoms in graphene carry magnetic moments μ ≈ μ B . In principle, the latter is not exceptional because defects and impurities in crystals without any d or f elements may have unpaired electrons and, therefore, exhibit paramagnetism [10] , [11] . However, achieving ferromagnetic alignment between these unpaired spins has proven practically impossible [10] . In graphene, the prospect of defect ferromagnetism is more realistic because, first, the presence of conduction electrons provides a medium for coupling between localized spins and, second, the defect-induced moments are believed to be due to the same π electrons that are responsible for electron transport [12] , [13] , [14] , [15] , [16] , [17] , [18] , [19] , [20] , [21] . Accordingly, it should be possible to use the electric-field effect to control not only the coupling between localized magnetic moments in graphene but also the presence of the moments themselves which so far has not been possible in other materials. In this contribution, we have employed Superconducting Quantum Interference Device (SQUID) magnetometry and molecular doping to investigate graphene’s paramagnetism. We have found that magnetic moments due to vacancies and adatoms can be switched off by shifting the Fermi energy E F above ≈0.45 eV and then switched back on by returning to the neutral state or lower E F . This proves the itinerant nature of magnetic moments in graphene, that is, π magnetism. The localization radius r L for the itinerant spins is estimated as ≈2.0 nm. For the case of vacancies, we find them carrying two practically independent moments that are attributed to the π magnetism and an unpaired spin on broken bonds. Only half of vacancy magnetism can be switched off by doping. A profound implication of our findings is that π magnetism can be controlled by other means, notably by the electric field doping within realistically accessible carrier densities n ≈2 × 10 13 cm −2 . Furthermore, it is likely that the unexpectedly quick spin relaxation found in graphene devices and attributed to magnetic defects [22] can be quenched by doping above the above threshold. Magnetic response of graphene with vacancies Our samples were graphene laminates that were shown [8] to be a well-characterized, clean reference system, providing enough material (typically, several mg of graphene) for SQUID magnetometry. Our magnetometer (Quantum Design MPMS XL7) allowed measurements at temperatures T between 300 and 1.8 K in fields H up to 7T. The samples were irradiated with 350 keV protons to achieve the desired density of single vacancies, n v (Methods). Irradiation resulted in a pronounced paramagnetic response arising from non-interacting moments [8] . Typical magnetization curves are shown in Fig. 1 . For all vacancy concentrations, such curves were accurately described by the Brillouin function with spin S =1/2. The measured magnetic moment M was found to be proportional to n v as M , where μ B is the Bohr magneton and N S is the number of spins extracted from Brillouin function fits, in agreement with the earlier report [8] . 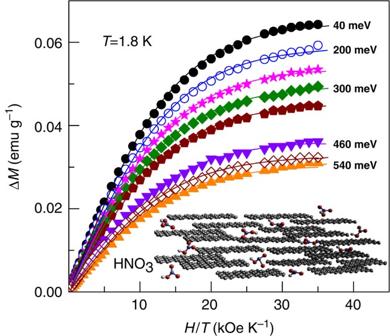Figure 1: Effect of hole concentration on vacancy paramagnetism. Symbols show the measured magnetic moment ΔMas a function of magnetic fieldHfor different hole concentrationsn. A linear diamagnetic background is subtracted (Methods). Solid curves are fits to the Brillouin function withS=1/2. Labels show the corresponding Fermi energy |EF| in the valence band. Inset: Illustration of HNO3molecules physisorbed in graphene laminates. Figure 1: Effect of hole concentration on vacancy paramagnetism. Symbols show the measured magnetic moment Δ M as a function of magnetic field H for different hole concentrations n . A linear diamagnetic background is subtracted (Methods). Solid curves are fits to the Brillouin function with S =1/2. Labels show the corresponding Fermi energy | E F | in the valence band. Inset: Illustration of HNO 3 molecules physisorbed in graphene laminates. Full size image Control of carrier concentration in graphene laminates To probe the evolution of M as the valence (conduction) band gets progressively filled up with holes (electrons), we varied the carrier concentration by using molecular doping: nitric acid (HNO 3 ) or NO 2 gas as hole dopants [23] , [24] , [25] and aniline as an electron dopant [26] . The properties of HNO 3 and NO 2 as acceptors were investigated both theoretically [24] and experimentally [23] , [25] , and both were shown to be very effective, with each physisorbed molecule resulting in transfer of one electron [25] (see Methods for details). However, finding an effective donor turned out to be problematic. Aniline is reported as one of the best donors but the maximum doping it allowed was only n ≈5 × 10 12 cm −2 . Within the limited range of n achievable for aniline, we have found no difference with respect to hole doping with HNO 3 and, therefore, focus below on the latter results. Effect of doping on magnetization of irradiated graphene Figure 1 shows the evolution of M ( H ) curves for one of the irradiated samples as it is doped from a nearly neutral state to E F ≈0.5 eV. It is clear that the doping has a strong effect on magnetization: M reduces to half its initial value, even though all M ( H ) curves look qualitatively the same and are accurately described by the Brillouin function with S =1/2. This indicates a reduction in the number of magnetic moments for the same number of vacancies. It also shows that high n do not lead to stronger interaction, as the vacancy magnetic moments remain noninteracting. This behaviour was found to be universal, even though n v varied for different samples by more than an order of magnitude, with the average separation between vacancies changing from ~3 to 10 nm. 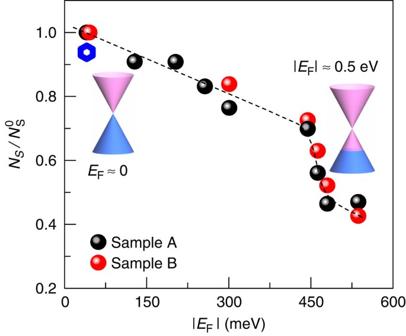Figure 2: Reversible control of vacancy magnetism. Normalized density of spins (S=1/2) in two irradiated samples as a function of their doping.is the spin concentration before doping8, andNSis extracted from the Brillouin function fit for theM(H)dependence for each doping level, whereMis the measured magnetization andHis the applied magnetic field. The dashed curve is a guide to the eye. Open symbol is for sample B after it was maximally doped and then annealed at ~100 °C for 2 h. The insets are schematic illustrations of the graphene spectrum in neutral and heavily doped states. Figure 2 shows the evolution of the number of detected spins N S in two graphene samples with different n v as a function of E F . Initially, N S is gradually decreasing with increasing the hole concentration, but at E F ≈0.4 eV, it falls sharply and seems to saturate to N S ≈ N S 0 /2 at the maximum doping, where N S 0 is the number of spins before doping. As soon as the dopants were removed from graphene by mild annealing, M recovered its initial value, that is, the effect is fully reversible ( Fig. 2 ). Figure 2: Reversible control of vacancy magnetism. Normalized density of spins ( S =1/2) in two irradiated samples as a function of their doping. is the spin concentration before doping [8] , and N S is extracted from the Brillouin function fit for the M(H) dependence for each doping level, where M is the measured magnetization and H is the applied magnetic field. The dashed curve is a guide to the eye. Open symbol is for sample B after it was maximally doped and then annealed at ~100 °C for 2 h. The insets are schematic illustrations of the graphene spectrum in neutral and heavily doped states. Full size image E F ≈0.54 eV was the maximum doping that we were able to achieve with HNO 3 , in agreement with the calculated energy dependence of the density of states (DOS) for the NO 2 molecule adsorbed on graphene [24] . The data scatter between different samples and doping levels does not allow us to follow the transition in Fig. 2 in more detail and confirm the apparent saturation to half magnetization above E F ≈0.45 eV. However, this behaviour was observed for many samples and repeatedly after annealing cycles. To gain further insight, Fig. 3 plots the reduction in magnetization signal at maximum doping, which was measured for several samples with different vacancy densities. It is clear that, independent of the sample and its N S 0 , the 50% reduction in M is universal, as long as the Fermi level is shifted sufficiently away from the neutrality point. 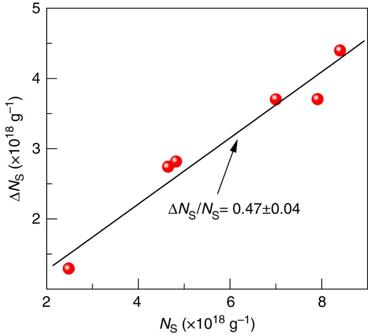Figure 3: Universal halving of the vacancy magnetic moment by doping. Symbols show the change in the number of spins after maximum doping,in samples with different vacancy concentrations,nv.is the spin concentration before doping andis the number of spins measured atEF≥0.5 eV. Solid line is the best fit ΔNS/NS0=0.47±0.04. Figure 3: Universal halving of the vacancy magnetic moment by doping. Symbols show the change in the number of spins after maximum doping, in samples with different vacancy concentrations, n v . is the spin concentration before doping and is the number of spins measured at E F ≥0.5 eV. Solid line is the best fit Δ N S / N S 0 =0.47±0.04. Full size image We attribute this finding to the presence of two types of magnetic moments associated with a vacancy, and only one of them is being affected by such a shift in E F . Indeed, let us recall the origin of defect-induced magnetism in graphene. It lies in the imbalance that the defects create between its two sublattices and the resulting appearance of localized π states with energy close to the Dirac point [12] , [13] , [14] , [15] , [16] , [17] , [18] , [19] , [20] , [21] . As long as these states are singly occupied, due to Coulomb repulsion, U C , they give rise to magnetic moments μ =1 μ B . This simple picture is expected for adatoms, such as fluorine or hydrogen, whereas for vacancies the origin of magnetic moments is more complex. In addition to the above π moments, there are dangling σ bonds that can have some role too [14] , [16] , [18] , [19] , [20] , [21] . For example, vacancies in insulating boron nitride are expected to be magnetic [27] . The relative contribution of σ states to vacancy magnetism is unknown and a matter of debate [18] , [20] . Because of high chemical reactivity of the dangling bonds, it is often assumed that they are saturated with, for example, hydrogen and therefore do not contribute to magnetism (see, for example, Palacios and Yndurain [18] and Nanda et al. [21] ). Then, the magnetic moment is purely due to itinerant (conduction) electrons. Another possible scenario is a vacancy reconstruction and the associated Jan–Teller distortion that results in hybridization between the π and σ states [14] , [19] , [20] , [21] . Depending on the degree of hybridization, the magnetic moment for a vacancy has been predicted to be between ~1.45 and 2 μ B [14] , [16] , [19] , [21] (refs14,16,19,21). Our experiment suggests an intermediate scenario in which the dangling bonds remain unsaturated and the hybridization does not have a significant role. In this case, each vacancy is expected to provide two independent contributions, which come from the singly occupied localized π state and the unsaturated σ bond. At sufficiently large doping, such that | E F |≥ U C , the localized π state becomes doubly occupied and the corresponding magnetic moment disappears, whereas the unpaired σ electron remains unaffected by doping and provides the residual M . Because the two contributions appear to be nearly equal, hybridization between the two electronic states should be weak. This is also in agreement with the measured S =1/2. Note that it would require unrealistically high doping to occupy the σ state and fully suppress the vacancy magnetism. To support the above interpretation, a neat experiment would be to compare the effect of doping on vacancy magnetism with that for adatoms, where there are no dangling bonds and only localized π states are expected [13] , [14] , [15] . However, it has proven difficult experimentally to introduce adatoms without their significant clustering. The latter locally opens a band gap, quenches nearest-neighbour magnetic moments and so on, so that the system can no longer be considered as graphene but becomes its chemical derivative [8] . We have circumvented this problem by exploiting the experimental fact that if graphene is heated at ≥350 °C, it results in the appearance of so-called resonant scatterers [28] , [29] , [30] , [31] . They reduce graphene’s electronic quality and result in the D peak in Raman spectra. The scatterers are attributed to some organic residue that is always present on graphene and strongly (sp 3 ) bonds to it at high T [28] . Resonant scatterers is another name for the localized π states near the Dirac point in the context of electron transport. With these earlier studies in mind, we annealed several samples of pristine (nonirradiated) graphene laminates at 350 °C in Ar–H 2 atmosphere. This induced notable paramagnetism with N S 0 ≈3 × 10 18 g −1 . The observed M ( H ) curves were practically identical to those of irradiated laminates and, again, are accurately described by the Brillouin function with S =1/2. The found N S 0 corresponds to 2–3 sp 3 bonds induced by annealing per each graphene crystallite in the laminates. In contrast to vacancy magnetism, the exposure of these sp 3 -defected samples to HNO 3 resulted in an almost complete disappearance of the paramagnetic signal above the same E F ≈0.45 eV ( Fig. 4 ), in agreement with expectations for the purely itinerant nature of sp 3 magnetism. Similar to the case of vacancies, the switching effect is also fully reversible: as soon as HNO 3 molecules were removed by mild annealing at ~100 °C, the paramagnetic signal recovered its initial value N S 0 . 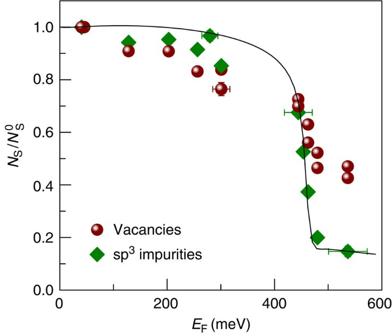Figure 4: Fully switchable π magnetism of adatoms. Comparison of the effect of doping on magnetism associated with vacancies (data fromFig. 2) and with sp3defects. Solid curve is the theoretical dependence of the normalized number of spins on the Fermi energy,NS/NS0(EF), calculated using equations (1) and (2), see text. Error bars indicate the accuracy of determination ofEF. Figure 4: Fully switchable π magnetism of adatoms. Comparison of the effect of doping on magnetism associated with vacancies (data from Fig. 2 ) and with sp 3 defects. Solid curve is the theoretical dependence of the normalized number of spins on the Fermi energy, N S / N S 0 ( E F ), calculated using equations (1) and (2), see text. Error bars indicate the accuracy of determination of E F . Full size image The magnetic moment due to sp 3 impurities and its variation with doping can be calculated analytically using the expression: which describes the DOS in graphene due to resonant scatterers such as sp 3 adsorbates (see Supplementary Note 1 ). Here, E d is the states’ energy position and a the hybridization parameter, both in units of the half width W ≈3 t of graphene’ energy band ( t is the nearest-neighbour hopping parameter). For sp 3 impurities relevant to our experiment (monovalent organic groups or hydrogen adatoms), E d =0.02 and a =2/3 (that is, hybridization strength ≈2 t ) [31] . The magnetic moment (number of spins) is given by the fraction of singly occupied impurity states, which is determined by the Hubbard energy U and can be found by integrating equation (1) over the occupied states: Using equation (2), we obtained the N S ( E F ) shown in Fig. 4 , which effectively has only one fitting parameter, U , because the dependence is found to be qualitatively insensitive to E d and a over a wide range of the parameters (the best-fitting value of U as in Fig. 4 is U =0.5 eV). N S drops sharply at E F ≈ U as expected, exhibiting a cusp-like dependence 1/ln| E F − U |. Note that the cut off does not lead to zero magnetization, which seems surprising but is in agreement with the experiment. The reason for a finite remaining N S on the theoretical curve is that the DOS deviates significantly from the standard Lorentzian peak. This arises due to the linear increase in the DOS of conduction electrons in graphene and a renormalization of the positions of impurity states because of hybridization. As a result, N ( E ) decays as 1/| E |ln 2 | E | at large E , much slower than the standard 1 /E 2 dependence for the Lorentz distribution. This means that the magnetic states become totally doubly occupied only for E F >> U and, therefore, N S exhibits a long tail at higher E F such as in Fig. 4 . Finally, let us add several comments. First, the found value of the Coulomb energy U =0.5 eV allows us to estimate the spatial localization r L of the π states as r L ≈2.0 nm (using the known effective Coulomb interactions in graphene [32] ), that is, the π state is localized over several benzene rings, in agreement with theory [13] , [14] , [16] . Second, comparing the nearly constant N S at E F <0.3 eV for sp 3 impurities in Fig. 4 (both theory and experiment) with gradually decreasing N S for vacancies indicates that the magnetic moment is sensitive to the shape of the DOS peak: the latter is much broader for vacancies [14] resulting in a more gradual decrease of N S in equation (2), in agreement with experiment. Third, an alternative mechanism for quenching of the magnetic moments at high n could be the Kondo effect [17] , [20] . However, the observed cumulative contribution from localized and itinerant moments and their T dependence ( Supplementary Figs S3 and S4 ) do not support this scenario (see Supplementary Note 2 ). Fourth, the discussed threshold doping is achievable in field-effect devices with high-quality gate dielectrics such as boron nitride. This should allow strong suppression of the rapid spin relaxation, characteristic to the existing graphene devices, so that spin currents can be efficiently switched on and off by gate voltage as required for a spin transistor operation. Preparation of irradiated graphene laminates Our graphene samples were prepared as described in Nair et al. [8] In brief, we used ultrasonic cleavage of highly oriented pyrolytic graphite in an organic solvent, N -methylpyrrolidone, following the procedure described in Sepioni et al. [33] The resulting laminates consist of predominantly 30–50 nm crystallites, aligned parallel to each other and electronically decoupled [8] . During filtration of the graphene suspension in N -methylpyrrolidone, the crystallites do not re-stack into graphite but remain rotationally disordered, with the average separation between graphene flakes ≈0.36 nm, significantly larger than the interplane distance in graphite. Vacancies were introduced by proton irradiation in a 500-kV ion implanter, at room temperature T and current density <0.2 μA cm −2 . The energy (between 350–400 keV), fluence (1.2–11 × 10 15 cm −2 ) and other irradiation parameters for each sample were chosen to achieve a desired defect density and ensure uniformity of defect distribution [8] . Proton irradiation under such conditions produces predominantly single vacancies [12] ; their number for each sample was estimated on the basis of the corresponding fluence, surface area and the number of defects created by each proton as obtained from computer simulations (SRIM software package). Further details can be found in Nair et al. [8] We note that impacts of energetic protons on graphene may also give rise to a finite concentration of other defects, such as divacancies and carbon adatoms, but their effect on magnetism is negligible, as the former do not possess magnetic moment and the latter are mobile at room temperature and tend to cluster with the loss of magnetism [34] . In our SQUID measurements, the field was usually applied parallel to the lamination direction to avoid diamagnetism that is strong in the perpendicular field [8] . A small remnant diamagnetic background due to some misalignment was linear with H up to 7T at all T and subtracted for clarity from the plotted data. Molecular doping and determination of carrier concentrations Molecular doping has been shown to be an effective way of changing carrier concentration in graphene, with water, NO 2 gas and HNO 3 identified as acceptors (hole dopants) and ammonia, anisole, aniline and N,N,N′,N′-tetramethyl-p-phenylenediamine (TMPD) as donors (electron dopants) [23] , [25] , [26] , [35] , [36] , [37] , [38] , [39] . After testing the above molecules on graphene laminates, HNO 3 was found to be the only molecule providing sufficiently high carrier concentrations, n (up to n ≈2 × 10 13 cm −2 , see below), excellent stability ( n remained same for several weeks) and uniform distribution (as manifested in same n measured in different locations on graphene laminates). To achieve gradual changes in n , the laminates were exposed to HNO 3 diluted with water at different molar concentrations of 0.1–15 M. The maximum doping level that we could achieve corresponded to n ≈2 × 10 13 cm −2 or . Importantly, once exposed to HNO 3 , the carrier concentration remained stable for many days at room T , in agreement with relatively high adsorption energy for this molecule [23] but recovered the initial value under mild annealing in argon. Gaseous NO 2 produced qualitatively similar results (in terms of both measured n and the effect on magnetization), but the doping level was difficult to control and showed significant nonuniformity. Ammonia did not produce any measurable permanent changes in n , presumably because of the difficulty in diffusing ammonia molecules between graphene layers and also much smaller adsorption energy compared with NO 2 [38] (ref. 38). The only donor that produced systematic changes in n was aniline [36] , but the maximum possible n was small (~5 × 10 12 cm −2 ) and resulted in only a small reduction in paramagnetic magnetization, similar to the effect of hole doping at such n . Another known electron dopant N,N,N′,N′-tetramethyl-p-phenylenediamine (TMPD) [39] was found to exhibit weak paramagnetism of its own and, therefore, was avoided. To monitor the changes in n , we used Hall effect measurements (see Supplementary Fig. S1 ). They were done on 3 × 3 mm 2 samples cut out of a 2-cm diameter laminate obtained after filtration. The concentration was calculated as n = I·B /( V H · e·N l ), where I is the applied current, B is the magnetic field, V H is the Hall voltage and N l is the number of graphene layers in the laminate. The latter was calculated from the measured sample thickness, typically 3–5 μm, and the average separation between the layers d ≈0.36 nm, as determined using X-ray diffraction. In addition to the Hall measurements, we used Raman spectroscopy that is also sensitive to n [25] , [40] , [41] (refs 25,40,41). Raman measurements were carried out using a Renishaw spectrometer with a green laser. As graphene crystallites in the laminates are small (typically 30–50 nm), they produce a significant broadening of all Raman peaks, which makes it difficult to detect exact shifts in their positions that would otherwise yield n . Therefore, we used graphene mechanically exfoliated onto Si/SiO 2 and treated these samples in parallel with graphene laminates used for the Hall and magnetization measurements. Raman spectroscopy on such isolated samples was found to be sufficiently sensitive to detect changes in n even for small changes in HNO 3 concentration. Examples of Raman spectra after exposure to different concentrations of HNO 3 are shown in Supplementary Fig. S2 . We examined the shift and intensity variations of the G peak that is most sensitive to n [25] , [40] , [41] . The changes were translated into n by using the calibration data for gated graphene [41] . The absence of the D peak either before or after exposure to HNO 3 (not shown) confirmed that HNO 3 molecules were physisorbed on graphene and not chemisorbed, as the D peak is known to be a measure of short-range defects such as sp 3 bonds [42] . Corresponding Fermi energies for each n were calculated using the relation E F =(π n ) 1/2 ħ v F , where v F =1.1 × 10 6 ms −1 is the Fermi velocity. We emphasize that the results, shown in Supplementary Fig. S2 , are in good agreement with the concentrations obtained from our Hall measurements for the same exposure to HNO 3 . As a further check, we also measured Raman spectra directly on graphene laminates at high doping (HNO 3 concentrations of 11–15 M), where the shift in the G peak position was sufficiently large (peak at 1600–1605, cm −1 ) to overcome the broadening effect. Again, the results were consistent with the Hall measurements and with the values of n obtained from the Raman spectra on exfoliated monolayers. For these particular measurements, the extracted values of n were in a range of 1–2 × 10 13 cm −2 . How to cite this article: Nair, R. R. et al. Dual origin of defect magnetism in graphene and its reversible switching by molecular doping. Nat. Commun. 4:2010 doi: 10.1038/ncomms3010 (2013).